Enantioselective Cu-catalyzed double hydroboration of alkynes to access chiral gem-diborylalkanes Chiral organoborons are of great value in asymmetric synthesis, functional materials, and medicinal chemistry. The development of chiral bis(boryl) alkanes, especially optically enriched 1,1-diboron compounds, has been greatly inhibited by the lack of direct synthetic protocols. Therefore, it is very challenging to develop a simple and effective strategy to obtain chiral 1,1-diborylalkanes. Herein, we develop an enantioselective copper-catalyzed cascade double hydroboration of terminal alkynes and highly enantioenriched gem -diborylalkanes were readily obtained. Our strategy uses simple terminal alkynes and two different boranes to construct valuable chiral gem -bis(boryl) alkanes with one catalytic and one ligand pattern, which represents the simplest and most straightforward strategy for constructing such chiral gem -diborons. Chiral organoborons are of great value in asymmetric synthesis and functional materials as well as bioactive molecules [1] , [2] , [3] , [4] , [5] , [6] , [7] , [8] . Myriads of protocols have been developed to construct chiral mono-organoborons with carbon-stereogenic centers [9] , [10] , [11] , [12] , [13] , which have been proven to be very valuable chiral building blocks in organic synthesis [14] , [15] . Compared with chiral mono-organoboron compounds, enantioenriched bis(boryl) ones might provide the feasibility for selective and multiple C-C or C-heteroatom bonds constructions to generate new valuable chiral compounds. However, chiral bis(boryl) compounds are underdeveloped due to the paucity of straightforward synthetic strategies. The development of efficient synthetic protocols to access various chiral bis(boryl)alkanes is highly desirable for investigating their fundamental properties and exploring their potential applications. Enantioselective hydroboration of widely existing alkenes is one of most important and efficient means to construct chiral organoboron compounds, yet which usually only leads to chiral mono-organoborons, sequential double hydroboration of readily available alkynes was considered as one of the most ideal strategies for synthesizing bis(boryl)alkanes, however, because of the inherent challenges on controlling the chemo-, regio-, and enantioselectivities on the hydrofunctionalizations of alkynes and multicomponent reactions, enantioenriched double hydroborations of alkynes have been scarcely reported [9] , [10] , [11] , [12] , [13] . In 2009, Hoveyda presented an enantioselective copper-catalyzed 1,2-hydroboration of aliphatic terminal alkynes for the synthesis of 1,2-bis(boryl) alkanes with B 2 pin 2 as boron source and MeOH as hydrogen donor [16] ; in 2012, Yun and coworkers disclosed a highly regio- and stereoselective Cu-catalyzed double hydroboration of silylalkynes to render syn -vicinal diboronates, once again with B 2 pin 2 /MeOH system [13] . Compared to enantioselective 1,2-double hydroboration of alkynes, chiral 1,1-diborylalkanes which contain two different boryl units on the same carbon atom are very rare, the seminal example came from the Hall group in 2011 [17] , in which chiral 1,1-diborons were generated from enantioselective Cu-catalyzed hydroboration of alkenylBdan substrates (dan, 1,8-diaminonaphthalenyl-) with B 2 pin 2 as boron source. Two years later, Yun and coworkers disclosed an enantioselective hydroboration of alkenylBdan via Cu-catalysis with HBpin as boron source (Fig. 1A ) [2] . Despite as the sporadic seminal two methods on the preparation of chiral 1,1-diboryl alkanes, Hall’s strategy and Yun’s method have significant shortcomings, including the requirement to prepare the alkenylBdan as starting material through a one- or two-step synthesis, narrow substrate scope with very few examples, and limited synthetic applications employed for the chiral 1,1-diboryl alkanes. Recently, the Chirik group developed an asymmetric hydrogenation of unsymmetric 1,1-diboryl alkenes to render chiral 1,1-diboryl alkanes (Fig. 1B ) [18] . Once again, the starting materials in this strategy have to be presynthesized from alkynes and the chiral cobalt complexes are presynthesized as well. Given the prevalence and ready accessibility of alkynes and the principals of green chemistry on trimming down the synthetic steps, we envision alkynes could be a very good starting point for the construction of chiral 1,1-diboryl alkanes based on our previous experience on the synthesis of racemic 1,1-diborons. In order to build the optically pure 1,1-diborons, transition-metal catalyzed hydroboration of alkynes with HBR 2 as both boron source and hydrogen source should be the ideal solution for this goal. However, there are several significant challenges in our proposed protocols: mono-hydroboration might be the dominant one [19] ; homo-diboration might occur and will be a trouble for purification [20] , [21] ; regioselectivity is always an issue on the functionalization of alkynes [22] ; last but not the least, the stereocontrol will be a great challenge to surpass with suitable metal catalyst and appropriate chiral ligands. Our previous experience on transition metal-free multi-functionalization of alkynes [23] , [24] , [25] , [26] , [27] , [28] , [29] , [30] , [31] , [32] , [33] and cobalt-catalyzed cascade hydrosilylation and hydroboration of alkynes to access enantioenriched 1,1-silylboryl alkanes (Fig. 1C ) [34] led to speculation that the incorporation of transition metal with appropriate choice of double hydroboration partners will be crucial to overcome the aforementioned issues. Fig. 1: Enantioselective approaches to access chiral bis(boryl)alkanes. A Enantioselective hydroboration of alkenylBdan to chiral 1,1-diborons. B Asymmetric hydrogenation of 1,1-diboryl alkenes to chiral 1,1-diboryl alkanes. C Enantioselective Co-catalyzed hydrosilylation and hydroboration of alkynes to chiral 1,1-silyboronates (our previous work). D Our strategy for enantioselective copper-catalyzed double hydroboration of alkynes to chiral 1,1-diborons (this work). Full size image Here, we show a general and efficient strategy to construct enantioenriched 1,1-diboryl alkanes via a cascade copper-catalyzed double hydroborations of readily available alkynes (Fig. 1D ). The strategy offers a straightforward method and great value in streamlining access to the important chiral 1,1-diboryl alkanes in a manner that complements the existing method. This system takes advantage of the in situ formation of the key terminal alkenylBdan intermediate, followed by second enantioenriched hydroboration with HBpin (Bpin, pinacolato) with two steps sharing one catalytic system. This reaction is compatible with terminal alkynes with a variety of substituents (including aliphatic and aromatic ones) [35] , [36] , [37] , [38] , [39] and demonstrates high regio- and stereoselectivity during diborylations. Further mechanistic studies and DFT calculations help us to gain insights on the mechanism of beautiful regio- and stereoselectivity. Optimization studies of racemic process Our studies began to investigate the reaction of racemic process by using 4-phenyl-1-butyne ( 1 ) as the testing substrate. 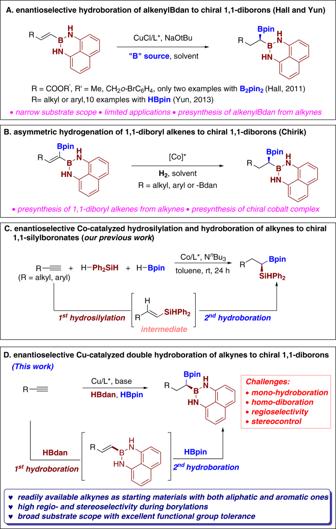Fig. 1: Enantioselective approaches to access chiral bis(boryl)alkanes. AEnantioselective hydroboration of alkenylBdan to chiral 1,1-diborons.BAsymmetric hydrogenation of 1,1-diboryl alkenes to chiral 1,1-diboryl alkanes.CEnantioselective Co-catalyzed hydrosilylation and hydroboration of alkynes to chiral 1,1-silyboronates (our previous work).DOur strategy for enantioselective copper-catalyzed double hydroboration of alkynes to chiral 1,1-diborons (this work). A series of conditions with 2,3-dihydro-1H-naphtho[1,8-de][1–3]diazaborinine (HBdan) as the borylation source, pinacolborane (HBpin) as another borylation reagent, NEt 3 as the base, Co(acac) 2 as catalyst and Xantphos as ligand were examined, which was successfully rendering 68% yield of target product 4 (Table 1 , entry 1). Subsequently, various metal catalysts were investigated, Co(acac) 2 emerged as the optimal catalyst (Table 1 , entries 2-3). After exploration of the other parameters like ligands, solvents and additives, the concentration of the reaction and the reactants adding-orders (Table 1 , entries 4-10, also see Supplementary Tables 1 to 5 for details), the best reaction conditions were identified as 0.2 mmol of alkyne, 0.24 mmol of HBdan, 0.6 mmol of HBpin, 4 mol % of Co(acac) 2 , 4 mol% of Xantphos and 3.0 equiv of NEt 3 in 0.2 mL of cyclohexane for 12 h (Table 1 , entry 9). Table 1 Discovery and parameter evaluation of the Co-catalyzed racemic cascade reaction a,b . Full size table Substrate scope for racemic process Achieving the optimal conditions with non-chiral transformation, we started to evaluate the universality of the optimized conditions (Table 1 , entry 9) in preparing racemic 1,1-diborons, the substrate scope was illustrated Fig. 2 . Various unactivated aliphatic or aromatic alkynes were investigated to afford the corresponding racemic 1,1-diborons with ideal reaction outcomes. The molecular structure of diboron 4 was confirmed by X-ray crystallographic analysis (CCDC 2039502, see Supplementary Fig. 15 for details). The influence of different carbon chain length of aliphatic alkynes was studied and the products 4 – 14 were obtained in decent yields respectively. The substrates bearing bulky isopropyl and cycloalkyl groups were also good candidates to deliver the targeted products in satisfactory yields ( 6 , 8 ). Alkynes which bear various functional groups, such as silyl-protected alcohol, diethoxypropyl, and ester were all compatible and the respective products ( 15 – 16, 18 – 33 ) were obtained in good yields. It is worthwhile to find that N -Boc-4-ethynylpiperidine can also react smoothly under our standard conditions ( 17 ). Of note, the olefin moiety ( 18 ) does not interfere with the reaction and remains intact, indicating that the reaction has good chemical selectivity and ideal regional selectivity. High functional compatibility forced us to extrapolate our strategy to bioactive or therapeutic agents (Fig. 2 ). Various bioactive molecules or medicinal agents were derived into the corresponding aliphatic alkynes, all of them could render the respective targeted products in very good response under our standard conditions (for instance, sorbic acid ( 22 ), 2-propylpentanoic acid ( 23 ), 1-phenylcyclopentane-1-carboxylic acid ( 24 ), (R)-2-phenylpropanoic acid ( 25 ), benzoic acid ( 26 ), (S)-ibuprofen ( 27 ), α-methylcinnamic acid ( 28 ), (1 S,2 S,4 R)-5-norbornene-2-carboxylic acid ( 29 ), 1,4-benzodioxan-2-carboxylic acid ( 30 ), adapalene ( 31 ), naproxene ( 32 ) and gemfibrozil ( 33 )). Gratifyingly, C-C double bond could well retain in our system, which also proved that this method has excellent chemoselectivity ( 22 , 28 and 29 ). Fig. 2: Scope of the racemic reaction a . Reaction conditions: a After Co(acac) 2 (4 mol%), Xantphos (4 mol%), HBdan (0.24 mmol) and NEt 3 (0.6 mmol) were mixed in cyclohexane (0.2 mL, 1 M) at room temperature for 10 min, HBpin (0.3 mmol) and 1 (0.2 mmol) were added subsequently at room temperature, then the resulting mixture was stirred at ambient temperature for 12 h. b 50 °C. Full size image Not only aliphatic terminal alkynes gave very good response, the double hydroborations could also apply to versatile aromatic acetylenes. Overall, the standard conditions tolerated both electron-rich and electron-deficient functional groups on the aromatic rings (Fig. 2 , bottom). When the aromatic ring bearing different substituents like Me, Et, t Bu, i Pr, C 4 H 9 , C 3 H 7 , Ph, OMe, OC 5 H 11 , NMe 2 , COOEt, the reaction could proceed smoothly and the expected products 35 – 46 were obtained in decent yields. It is noteworthy that the lower yields afforded in reactions with aryl alkynes bearing halogens on the para position, such substrates could be rectified by increasing the reaction temperature to 50 °C ( 47 – 53 ). Moreover, alkynes bearing other aromatic substituents such as dimethylthiochroman ( 54 ), thiophene ( 55 ), phenanthrene ( 56 ), 4-carbazolebenzene ( 57 ) and 2-naphthyl ( 58 ) were good candidates as well, rendering the targeted products in nice yields. Optimization studies of asymmetric process Inspired by the success in racemic synthesis of 1,1-diborons, we decided to interprete this racemic transformation to an enantioselective process. Initially, we used Co(acac) 2 as the catalyst and evaluated the chiral diphosphine ligands, and it turned out that Walphos was the best one by a series of trials. However, after extensively screening, we still struggled the low yields and unsatisfactory ee values. 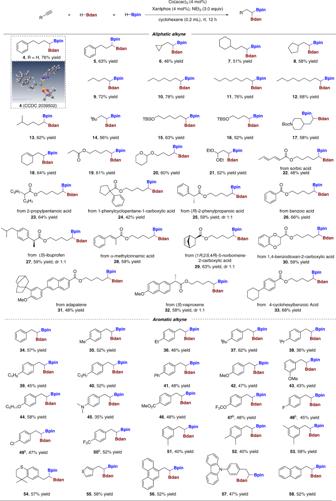Fig. 2: Scope of the racemic reactiona. Reaction conditions:aAfter Co(acac)2(4 mol%), Xantphos (4 mol%), HBdan (0.24 mmol) and NEt3(0.6 mmol) were mixed in cyclohexane (0.2 mL, 1 M) at room temperature for 10 min, HBpin (0.3 mmol) and1(0.2 mmol) were added subsequently at room temperature, then the resulting mixture was stirred at ambient temperature for 12 h.b50 °C. Given the influence of metals on the reaction outcomes, we decided to reevaluate metal catalysts (such as Co(acac) 2 , Co(acac) 3 , Cu(acac) 2 )., we were pleasantly surprised that Cu(acac) 2 could provide the optimal result with the enantioenriched 1,1-diborons 59 in 76:24 er (Table 2 , entry 4). Encouraged by the desired performance of Xantphos in reactions above, a series of structurally relevant chiral diphosphine ligands were investigated (Table 2 , entries 4-8, see Supplementary Table 8 for more details), whereas (R,R)-Me-Duphos and (R,R)-Me-Ferrocelane were found to be ineffective to our reaction (Table 2 , entries 7-8). After screening a series of solvents (see Supplementary Table 9 for details), no better results were obtained than cyclohexane (1.0 mL) (Table 2 , entry 9). After determining the best solvent, we screened the (R,R)-Walphos with different substitutions, and found that (R,R)-Walphos was still the best ligand. Then we did more research and testing about additives, the amount of catalysis and ligands, different adding-ordering and reaction time (see Supplementary Tables 10 , 13 and 14 for details). Table 2 Discovery and evaluation of the Cu-catalyzed asymmetric cascade process a . Full size table We found the reaction in the absence of PMHS, and the desired product could be obtained as well, however the yield and ee value were not satisfactory (33% yield with 88:12 er). Inspired by Engle’s work [10] , we studied the amount of PMHS and other base (see Supplementary Table 11 for details), and we found that the addition of PMHS is very important to the success of our transformation, and one equivalent of PMHS is required in order to get good yield of product, however, PMHS has little influence on the selectivity of our transformation [40] . Based on our previous work (Fig. 1C ) [34] , we realized that the sequence and the adding time will influence the efficiency of the transformation, therefore, we performed control experiments careful to figure out the length of adding time (see Supplementary Table 15 for details). It clearly demonstrated the importance of the time control in this transformation, and 10 mins after HBdan and PMHS addition with catalyst and ligand led to desired product with both good yield and good enantioselectivity. We think that the result might stem from the initial formation of Cu-H species from Cu catalyst and HBdan and PMHS. Further DFT calculations also suggest that the formation of intermediate alkenyl-Bdan is very important, otherwise, 1,1-diBpin will be an inevitable byproduct which origins from the intermediate alkenyl-Bpin, therefore, the addition of HBdan prior to HBpin is crucial to the good yields and enantioselectivity. Finally, we identified the best conditions as: After Cu(acac) 2 (6 mol%), Walphos (6 mol%), HBdan (0.24 mmol) and PMHS (1.0 equiv) were mixed in 1.0 mL of cyclohexane at room temperature for 10 min, HBpin (0.3 mmol) and 1 (0.2 mmol) were added subsequently at room temperature, then the resulting mixture was stirred at ambient temperature for 60 h. The desired chiral product 59 was obtained in 78% yield with 94:6 er (Table 2 , entry 14). Substrate scope in asymmetric transformation Having established the conditions for enantioselective reaction, we began to examine the reaction range and the results were depicted in Fig. 3 . To our delight, like their racemic congeners, various unactivated aliphatic and aromatic alkynes were investigated and smoothly deliver the corresponding chiral 1,1-diborons with desired reaction outcomes. Aliphatic alkynes with different carbon chain length were also examined to afford the desired products in good yields with high levels of stereoinduction ( 59 – 70 ). The molecular structure of asymmetric diboron 59 was confirmed by X-ray crystallographic analysis (CCDC 2107254, see Supplementary Fig. 16 for details). Of note, this asymmetric reaction could tolerate a variety of functionalities installed on the carbon chain such as Boc-protected amine ( 71 ), silyl-protected alcohol ( 72 – 75 ) and esters ( 76 – 87 ), this high functionality compatibility encouraged us to expand our synthetic scheme to the late stage elaborations of bioactive or pharmaceutic agents. Upon treatment with the standard conditions, a series of alkynes derived from sorbic acid, 2-propylpentanoic acid, benzoic acid, p -toluic acid, 4-cyclohexylbenzoic acid, α-methylcpiinnamic, gemfibrozil, (R)-2-phenylpropanoic acid, (S)-ibuprofen, (S)-naproxen and (1 S,2 S,4 R)-5-norbornene-2-carboxylic acid all rendered corresponding enantioenriched chiral gem -diborylalkanes in decent yields with both high regio- and stereoselectivities ( 77 – 86 ). The successful elaborations of these bioactive or therapeutic agents certified the mildness and broad functional group compatibility of this asymmetric transformation. Fig. 3: Scope of the chiral reaction a . Reaction conditions: a After Cu(acac) 2 (6 mol%), Walphos (6 mol%), HBdan (0.24 mmol) and PMHS (0.2 mmol) were mixed in cyclohexane (1.0 mL) at room temperature for 10 min, HBpin (0.3 mmol) and 1 (0.2 mmol) were added subsequently at room temperature, then the resulting mixture was stirred at ambient temperature for 60 h. b Josiphos (6 mol%). Full size image Of note, compared with the insensitivity to structural variation for aliphatic alkynes on enantioselectivity in the asymmetric conditions, aryl alkynes varied significantly. When we use phenylacetylene as substrate under the aforementioned standard condition, we can only achieve the target product 87 in 43% yield and 71:29 er. Through a series of optimization studies of process, we identified Josiphos as the best chiral diphosphine ligand which could provide 52% yield and 91:9 er in target product 87 . The molecular structure of asymmetric diboron 89 was confirmed by X-ray crystallographic analysis (CCDC 2118336, see Supplementary Fig. 17 for details). Chiral functionalized products with Me, Et, C 3 H 7 and substituents were prepared in useful yields and good er values ( 88 – 91 ). Mechanistic studies Since our experimental results show that the reaction is advantageous to the formation of 1,1- bifunctionalized product over other byproducts, we then studied the origin of significant regioselectivity and stereoselectivity in this transformation. When 1 was subjected to HBdan in the absence of HBpin, trace amount of alkenyl-Bdan 93 was detected by gas chromatography (GC) analysis with dodecane as internal standard under the standard reaction conditions (Fig. 4 , eq. 1). Of note, when only HBpin was added, 1,1-diboron alkane 94 was detected in 40% yield by GC analysis, meanwhile, alkyl Bpin 95 was detected with trace amount of alkenyl-Bpin 96 (Fig. 4 , eq. 2). Moreover, where HBdan, HBpin and alkyne were added simultaneously at the beginning of reaction, the target product 59 was detected in 53% yield with 90:10 er with 15% yield of 1,1-diboron alkane 94 detected (Fig. 4 , eq. 3). These outcomes indicated two feasible routes, that is whether alkenyl-Bdan 93 or alkenyl-Bpin 96 was built first for our transformation. To figure out the plausible pathway, we prepared the two possible intermediates alkenyl-Bdan 93 and alkenyl-Bpin 96 using the standard conditions for asymmetric synthesis. Under chiral standard conditions, alkenyl-Bdan 93 reacted with HBpin smoothly to afford 59 in 88% yield and 95:5 er (Fig. 4 , eq. 4a) but the reaction of alkenyl Bpin 96 with HBdan only in 14% yield and 44:56 er to give diboron product 59 (Fig. 4 , eq. 5a). When exposed to the racemic standard conditions, similar results were obtained: alkenyl-Bdan 93 reacted with HBpin smoothly to afford 4 in 86% yield (Fig. 4 , eq. 4b) but the reaction of alkenyl-Bpin 96 with HBdan did not proceed and only afforded trace amount of targeted product 4 (Fig. 4 , eq. 5b). Exposure of 59 under basic conditions in the presence of a large excess of CD 3 OD (0.5 mL) led to the selective protodeboration of the Bpin moiety, affording the Bdan-substituted alkane 97 in 74% yield and 99% D (Fig. 4 , eq. 6) [41] . Fig. 4: Control experiments. (1) 1 was exposed to HBdan in the absence of HBpin, under the standard reaction conditions. (2) 1 was exposed to HBpin in the absence of HBdan, under the standard reaction conditions. (3) One-pot reaction to the target product 59 . (4) alkenyl-Bdan 93 and HBpin was exposed under the standard reaction conditions. (5) alkenyl-Bpin 96 and HBdan was exposed under the standard reaction conditions. (6) Deuterium experiment. (7) the yield changes of alkenyl-Bdan 93 and targeted product 4 over the reaction time. Full size image Mechanistic investigations According to the previous report [2] , [9] , [10] , [11] , [12] , [16] , [13] , [17] , [18] , [19] , [40] , [42] , [43] , [44] and control experiments, we put forward the possible reaction mechanism about the copper-catalyzed enantioselective double hydroboration of alkynes (Fig. 5 ). The first hydroboration is started with the formation of copper hydride species from Cu(acac) 2 , ligand, HBdan and PMHS. Alkyne 1 reacts with the copper hydride species by Cu–H bond insertion to generate vinyl copper species I , which undertakes a σ-bond metathesis with HBdan to deliver vinyl Bdan II and release Cu-H species for finishing the first cycle and starting the second catalytic cycle. Vinyl Bdan II reacts with Cu–H species once again to generate alkyl copper species III , which further undertakes σ-bond metathesis with HBpin. The release of product IV and regeneration of Cu–H complex fulfill the catalytic cycle for the second hydroboration. Fig. 5: The proposed mechanisms. The reaction proceeds through 1 st hydroboration cycle with HBdan and 2 nd hydroboration cycle with HBpin. Full size image We next performed density functional theory (DFT) calculations to further validate our proposed mechanism (SMD-M06L/6-311+G(d,p)/SDD(Cu,Fe)//B3LYP-D3/6-31G(d)/SDD(Cu,Fe), computational details can be found in the Supplementary information 1 ). The structurally simplest cyclopropyl alkyne was chosen as the model substrate and the results are shown in Fig. 6 . The hydroboration cycles begin with the coordination of the alkyne substrate to the copper hydride ( Cat ), which undergoes regioselective alkyne insertion into the Cu–H bond via a four-membered transition state (structure not shown here, see Supplementary Fig. 1 for details) to generate vinyl copper species Int-1 . The computed free energy of activation (Δ G ‡ ) for this step is 17.4 kcal/mol and the free energy of reaction (Δ G ) is -22.3 kcal/mol, in accordance with previous computational results [10] . 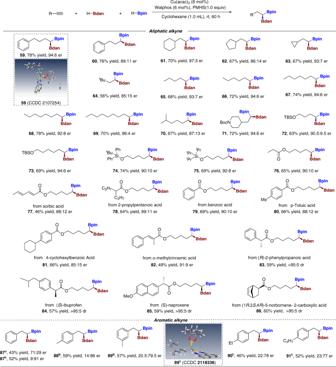Fig. 3: Scope of the chiral reactiona. Reaction conditions:aAfter Cu(acac)2(6 mol%), Walphos (6 mol%), HBdan (0.24 mmol) and PMHS (0.2 mmol) were mixed in cyclohexane (1.0 mL) at room temperature for 10 min, HBpin (0.3 mmol) and1(0.2 mmol) were added subsequently at room temperature, then the resulting mixture was stirred at ambient temperature for 60 h.bJosiphos (6 mol%). Int-1 could competatively react with H–Bdan 2 or H–Bpin 3 , undergoing either concerted or stepwise σ-bond metathesis processes via TS1 or TS5 to afford key alkenyl boron intermediates Int-2 or Int-6 , respectively, and regenerate the active copper hydride catalyst. Alkenyl Bdan Int-2 can subsequently react with the copper hydride catalyst ( Cat ) using either of its two faces (via TS2R or TS2S ) to generate chiral alkyl copper intermediates Int-3R or Int-3S , respectively. TS2R that ultimately leads to the major enantiomeric product ( R )- 63 is energetically favored than TS2S . Int-3R then undergoes chemoselective σ-bond metathesis with H–Bpin 3 via TS3R with retention of stereochemistry to furnish the catalytic cycle. The competing reaction of H–Bdan 2 with Int-3R via TS4 is higher in energy both kinetically and thermodynamically, in agreement with the experimental observation that Int-4 is not formed. In the competing pathway that initially forms alkenylBpin Int-6 , the subsequent 2 nd hydroboration favors the ultimate formation of 1,1-diboron species Int-8 via TS7 , which is the main side product observed experimentally. The reaction between Int-7 with H–Bdan 2 is disfavored with a much higher barrier and poor enantioselectivity. This result agrees well with the control experiment that the reaction between alkenyl boron 96 and H–Bdan 2 only afforded the corresponding product with 14% yield and 44:56 er. Overall, although the energies of the competing first hydroboration are comparable between alkenyl copper species Int-1 with H–Bpin 3 or H–Bdan 2 , its subsequent barrier via TS6S (18.0 kcal/mol) is higher than that of TS2R (10.6 kcal/mol). Taken together with the computed chemo- and enantioselectivities, and the results from the corresponding control experiments, the proposed mechanism for the formation of the main product is supported. The computational results also predicted the unavoidable formation of the side product, which rationalized the moderate yields of these reactions. To further probe the origin of the enantioselectivity for the hydrocupration process, we performed distortion/interaction analysis [45] on TS2R and TS2S (Fig. 6B ). The transition state structures were separated into two fragments that correspond to the Cu-H catalyst and the vinyl Bdan substrate, respectively. We found that the distortion energy of the catalyst (Δ E dist-cat ) is the main contributor to the enantioselectivity. The catalyst pocket accommodates one face of the approaching vinyl Bdan substrate better than the other. The relatively large and rigid structure of the planar Bdan group causes the phenyl group on the phosphine ligand to distort upwards in the disfavored TS2S , resulting in a larger distortion energy of the catalyst (10.8 kcal/mol) than that of TS2R (7.0 kcal/mol). Fig. 6: DFT calculations on the proposed reaction pathway. A Free energy profile for the competing hydroboration cycles. B Stereoselectivity-determining transition state structures. Full size image In summary, we disclose a Cu-catalyzed enantioselective 1,1-diboration reaction from two different boranes and readily accessible terminal alkynes. 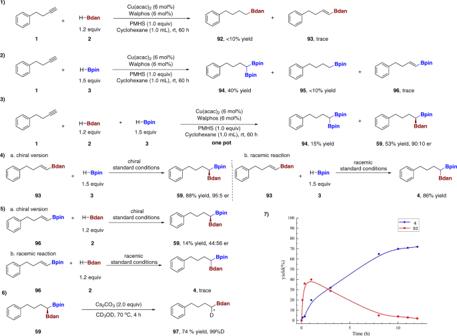Fig. 4: Control experiments. (1)1was exposed to HBdan in the absence of HBpin, under the standard reaction conditions. (2)1was exposed to HBpin in the absence of HBdan, under the standard reaction conditions. (3) One-pot reaction to the target product59. (4) alkenyl-Bdan93and HBpin was exposed under the standard reaction conditions. (5) alkenyl-Bpin96and HBdan was exposed under the standard reaction conditions. (6) Deuterium experiment. (7) the yield changes of alkenyl-Bdan93and targeted product4over the reaction time. This method demonstrates commendable regio-, chemo- and enantioselectivity, and could deliver valuable chiral gem -bis(boryl)alkanes with one catalysis and one ligand pattern from simple terminal alkynes and two different borane, which represents the most simple and straightforward strategy for the construction of such chiral gem -diborons. 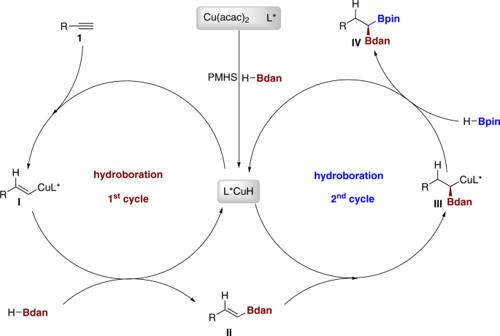Fig. 5: The proposed mechanisms. The reaction proceeds through 1sthydroboration cycle with HBdan and 2ndhydroboration cycle with HBpin. 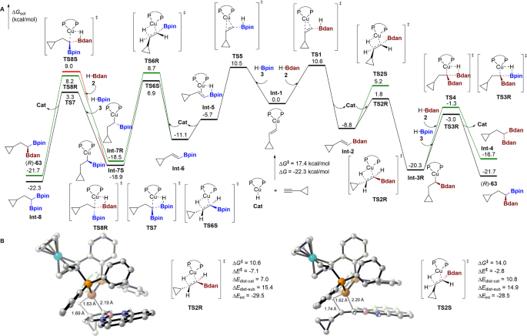Fig. 6: DFT calculations on the proposed reaction pathway. AFree energy profile for the competing hydroboration cycles.BStereoselectivity-determining transition state structures. We think that this research will encourage and intrigue efforts for the synthesis of derived enantioenriched borylalkanes, and provide new avenue for the asymmetric bifunctionalization of alkynes. DFT calculation illustrates the beautiful regioselectivity, chemoselectivity and enantioselectivity. General procedure A for synthesis of racemic gem -diborylalkane A tube was charged with Co(acac) 2 (4 mol%) and Xantphos (4 mol%) under N 2 atmosphere, then cyclohexane (0.2 mL), HBdan (0.24 mmol) and NEt 3 (0.6 mmol) were added subsequently. The reaction mixture was stirred at room temperature for 15 mins. Then HBpin (0.3 mmol) and 1 (0.2 mmol) were added subsequently at room temperature, then the resulting mixture was stirred at room temperature for 12 h. The residue was purified by column chromatography to afford the corresponding gem -diborylalkanes 4 . General procedure B for synthesis of racemic gem -diborylalkane A tube was charged with Co(acac) 2 (4 mol%) and Xantphos (4 mol%) under N 2 atmosphere, then cyclohexane (0.2 mL), HBdan (0.24 mmol) and NEt 3 (0.6 mmol) were added subsequently. The reaction mixture was stirred at room temperature for 15 mins. Then HBpin (0.3 mmol) and phenylacetylene containing halogen (0.2 mmol) were added subsequently at room temperature, then the resulting mixture was stirred at 50 °C for 12 h. The residue was purified by column chromatography to afford the corresponding product gem -diborylalkanes 47 . General procedure C for synthesis of chiral gem -diborylalkane A tube was charged with Cu(acac) 2 (6 mol%) and Walphos (6 mol%) under N 2 atmosphere, then cyclohexane (1.0 mL), HBdan (0.24 mmol) and PMHS (1.0 equiv) were added subsequently. The reaction mixture was stirred at room temperature for 10 mins. Then HBpin (0.3 mmol) and 1 (0.2 mmol) were added subsequently at room temperature, then the resulting mixture was stirred at ambient temperature for 60 h. The residue was purified by column chromatography to afford the corresponding product (R)-59 . General procedure D for synthesis of chiral gem -diborylalkane A tube was charged with Cu(acac) 2 (6 mol%) and Josiphos (6 mol%) under N 2 atmosphere, then cyclohexane (1.0 mL), HBdan (0.24 mmol) and PMHS (1.0 equiv) were added subsequently. The reaction mixture was stirred at room temperature for 10 mins. Then HBpin (0.3 mmol) and phenylacetylene (0.2 mmol) were added subsequently at room temperature, then the resulting mixture was stirred at ambient temperature for 60 h. The residue was purified by column chromatography to afford the corresponding product (S)-87 .